Non-hyperpolarizing GABABreceptor activation regulates neuronal migration and neurite growth and specification by cAMP/LKB1 γ-Aminobutyric acid is the principal inhibitory neurotransmitter in adults, acting through ionotropic chloride-permeable GABA A receptors (GABA A Rs), and metabotropic GABA B Rs coupled to calcium or potassium channels, and cyclic AMP signalling. During early development, γ-aminobutyric acid is the main neurotransmitter and is not hyperpolarizing, as GABA A R activation is depolarizing while GABA B Rs lack coupling to potassium channels. Despite extensive knowledge on GABA A Rs as key factors in neuronal development, the role of GABA B Rs remains unclear. Here we address GABA B R function during rat cortical development by in utero knockdown (short interfering RNA) of GABA B R in pyramidal-neuron progenitors. GABA B R short interfering RNA impairs neuronal migration and axon/dendrite morphological maturation by disrupting cyclic AMP signalling. Furthermore, GABA B R activation reduces cyclic AMP-dependent phosphorylation of LKB1, a kinase involved in neuronal polarization, and rescues LKB1 overexpression-induced defects in cortical development. Thus, non-hyperpolarizing activation of GABA B Rs during development promotes neuronal migration and morphological maturation by cyclic AMP/LKB1 signalling. γ-a-Aminobutyric acid (GABA) is the principal inhibitory neurotransmitter in the adult acting through ionotropic GABA A and metabotropic GABA B receptors (GABA A Rs, GABA B Rs) [1] , [2] . GABA A Rs are chloride-permeable channels. GABA B Rs are heterodimers of GABA B1 and GABA B2 subunits that operate through G proteins localized at pre- and post-synaptic sites. In particular, GABA B Rs are coupled presynaptically to Ca 2+ channels, regulating the release of neurotransmitters, and postsynaptically to K + inward rectifying (Kir) channels (Kir3), regulating postsynaptic slow inhibition [3] . Moreover, GABA B Rs also modulate cyclic AMP (cAMP) signalling, although the physiological consequences of this are poorly understood [3] . Interestingly, GABA does not mediate hyperpolarization-dependent inhibition during early development, as GABA A R signalling is mainly depolarizing and excitatory, and GABA B R lacks coupling between G proteins and Kir3 channels until the end of the first postnatal week [4] , [5] , [6] . Furthermore, abundant endogenous GABA present in neonatal tissue [1] , [2] , [6] , [7] activates GABA B Rs [8] . Despite the extensive literature on the importance of GABA A R during early development [1] , [2] , [6] , [7] , [9] , the role of GABA B R has been poorly investigated and data are controversial [10] . For example, a role of GABA B R in neuronal morphological maturation was described in some systems [9] , [11] , [12] , but not in others [13] , and only in vitro evidence indicated that GABA B R modulates migration of immature neurons [14] , [15] , [16] , [17] . Furthermore, these in vitro data are in contrast with observations in a number of mouse strains genetically modified for GABA B Rs, which present grossly normal brain and cell morphology [18] , [19] , [20] , [21] , [22] , [23] , [24] , [25] , [26] . Nevertheless, this may depend on compensatory mechanisms [6] . Here, to investigate GABA B R function during in vivo development, while avoiding compensatory mechanisms, we acutely downregulated GABA B2 subunit in a subpopulation of cortical pyramidal-neuron progenitors by in utero electroporation. We found that reducing GABA B2 -subunit expression results in impairment of cortical migration and morphological maturation of pyramidal neurons, through a mechanism dependent on cAMP signalling. GABA B2 short interfering RNA affects neuronal radial migration in vivo In rodents, glutamatergic neurons are generated in the dorsal ventricular and subventricular zones (VZ, SVZ) of the developing embryonic cortex. After acquisition of a bipolar morphology at the SVZ, these neurons migrate under the guidance of radial glia towards the developing cortical plate (CP), leading to the formation of the layered cortex [27] . Conversely, interneurons originate at the ganglionic eminence and migrate tangentially to the CP. Interestingly, GABA is more abundant at embryonic stage than at postnatal age [1] , [2] , [6] , [7] , as we confirmed in interneurons migrating tangentially in the lower intermediate zone (IZ) and in the neuropil ( Supplementary Fig. S1a,b ). Moreover, GABA B R is highly expressed at the SVZ and CP ( Supplementary Fig. S1c ) ( [8] ). To investigate the role of endogenous GABA B R during development in vivo , we used in utero electroporation of plasmids encoding small interfering RNA (short interfering RNA, siRNA) to interfere with GABA B -protein translation in a subpopulation of VZ/SVZ excitatory-neuron progenitors and their neuronal progeny. We prepared three short hairpin RNAs targeting the B 2 subunit of the GABA B R, and cloned them into the pRNAT-U6.3 expression vector, which drives expression of enhanced green fluorescent protein (EGFP) for visualization of transfected neurons ( Supplementary Fig. S2a–c ). siRNA1 and siRNA2 efficiently downregulated endogenous GABA B2 subunit with siRNA2 exhibiting higher efficiency ( Fig. 1a ; Supplementary Fig. S3a,b ). Moreover, whole-cell patch clamp recordings of GABA B2 -induced Kir currents demonstrated that siRNA2 efficiency lasted at least 1 month after electroporation ( Fig. 1c ). siRNAc did not produce any effect and was utilized (as the siRNA empty vector) as control ( Fig. 1a ). 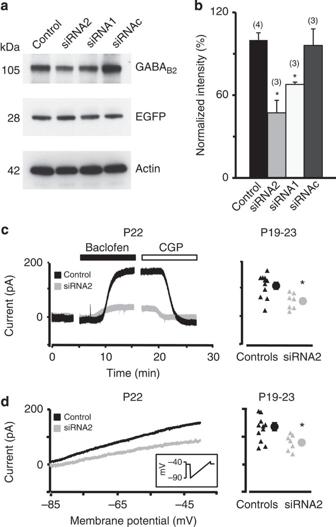Figure 1: GABAB2-siRNA allows long-lasting downregulation of endogenous GABAB2-subunit expression. (a) Western blot showing downregulation of GABAB2subunit in cortical neurons in culture at 3 DIV. Three siRNA duplexes (siRNA1, siRNA2 and siRNAc) were tested. Both siRNA1 and siRNA2 were effective in downregulating endogenous GABAB2expression (seeSupplementary Fig. S10). (b) Quantification of western blot experiments showing the level of GABAB2-subunit downregulation with the different siRNA duplexes, as ina. Data represent average value normalized to control (siRNA vector)±s.e.m. The asterisks indicate statistically significant difference compared with control (one-way ANOVA,P=0.003;post-hocHolm–Sidak method,P<0.05). Numbers in parentheses: number of independent transfections. (c) Examples of whole-cell patch clamp recordings of K+currents obtained during bath application of GABABR agonist (baclofen, 50 μM) and antagonist (CGP, 2 μM) in acute somatosensory cortical slices from control- (black) and siRNA2- (grey) transfected animals. K+currents were recorded in the presence of TTX (0.1 μM), kynurenic acid (1 mM) and bicuculline (2 μM) to block Na+channels, glutamate ionotropic receptors and GABAARs, respectively. Four weeks afterin uteroelectroporation, siRNA2-transfected cells were still exhibiting lower K+currents, indicating that siRNA2 was still transcribed and able to downregulate GABAB2-subunit expression. Right: quantification of all recorded K+currents. Triangles represent data from single cells and the circle represents the average±s.e.m., Data from siRNA2-transfected cells were statistically different (*) from controls (empty vector, WT cells; Student’st-test,P=0.008). (d) Examples of patch clamp recordings of inward rectifying K+currents (reduced current slope at depolarized membrane potentials) during a ramp test protocol (from −90 to −40 mV, 500 ms, inset) in conditions as inc. Peak Kir currents induced by baclofen were calculated as the peak of the trace obtained by the difference ofI-Vcurves before and after baclofen bath application, as already described22. Right: quantification of the peak amplitude of all recorded currents. Triangles represent data from single cells and the circle represents average±s.e.m. The asterisk indicates statistically significant difference compared with control (Student’st-test,P=0.016). Figure 1: GABA B2 -siRNA allows long-lasting downregulation of endogenous GABA B2 -subunit expression. ( a ) Western blot showing downregulation of GABA B2 subunit in cortical neurons in culture at 3 DIV. Three siRNA duplexes (siRNA1, siRNA2 and siRNAc) were tested. Both siRNA1 and siRNA2 were effective in downregulating endogenous GABA B2 expression (see Supplementary Fig. S10 ). ( b ) Quantification of western blot experiments showing the level of GABA B2 -subunit downregulation with the different siRNA duplexes, as in a . Data represent average value normalized to control (siRNA vector)±s.e.m. The asterisks indicate statistically significant difference compared with control (one-way ANOVA, P =0.003; post-hoc Holm–Sidak method, P <0.05). Numbers in parentheses: number of independent transfections. ( c ) Examples of whole-cell patch clamp recordings of K + currents obtained during bath application of GABA B R agonist (baclofen, 50 μM) and antagonist (CGP, 2 μM) in acute somatosensory cortical slices from control- (black) and siRNA2- (grey) transfected animals. K + currents were recorded in the presence of TTX (0.1 μM), kynurenic acid (1 mM) and bicuculline (2 μM) to block Na + channels, glutamate ionotropic receptors and GABA A Rs, respectively. Four weeks after in utero electroporation, siRNA2-transfected cells were still exhibiting lower K + currents, indicating that siRNA2 was still transcribed and able to downregulate GABA B2 -subunit expression. Right: quantification of all recorded K + currents. Triangles represent data from single cells and the circle represents the average±s.e.m., Data from siRNA2-transfected cells were statistically different (*) from controls (empty vector, WT cells; Student’s t -test, P =0.008). ( d ) Examples of patch clamp recordings of inward rectifying K + currents (reduced current slope at depolarized membrane potentials) during a ramp test protocol (from −90 to −40 mV, 500 ms, inset) in conditions as in c . Peak Kir currents induced by baclofen were calculated as the peak of the trace obtained by the difference of I-V curves before and after baclofen bath application, as already described [22] . Right: quantification of the peak amplitude of all recorded currents. Triangles represent data from single cells and the circle represents average±s.e.m. The asterisk indicates statistically significant difference compared with control (Student’s t -test, P =0.016). Full size image First, we examined the functional consequence of GABA B2 -subunit downregulation on cortical development by investigating the radial migration of newly generated excitatory cortical neurons. We injected either siRNA1 or siRNA2, or control vectors (siRNA vector or siRNAc), into the lateral ventricle of embryonic day 17 (E17) rats in utero , and electroporated them into a subpopulation of excitatory-neuron progenitors [28] . After allowing in vivo development, brains at E21, postnatal day 7 (P7), and P16 were cut at the level of the somatosensory cortex. As EGFP expression from the cytomegalovirus promoter in the pRNAT-U6.3 expression vector ( Supplementary Fig. S2a–c ) decreases with time in vivo , siRNA constructs were coelectroporated with pCAG-IRES-tdTomato vector (Tomato, Supplementary Fig. S2f ). Tomato vector bears a modified β-actin promoter with a cytomegalovirus immediate-early enhancer expressing a red fluorescence protein (tdTomato) ensuring visualization of transfected cells up to ~1 month ( [29] ). Confocal images of cortical neurons derived from siRNA-transfected progenitors were acquired by using tdTomato fluorescence, which strongly correlated (at E21) with EGFP (siRNA) fluorescence (Pearson product moment correlation, R =0.88±0.05; n =13 slices, Supplementary Fig. S4a,c ) in cells co-transfected in utero with siRNA and Tomato vectors ( Supplementary Fig. S2b,f ). Four days after electroporation (E21), control siRNA vector/Tomato-labelled cells in coronal slices were found mostly in the CP ( Fig. 2a ). However, radial migration in siRNA1/Tomato- and siRNA2/Tomato-electroporated animals appeared delayed, as transfected cells were found mostly in the IZ ( Fig. 2a ). 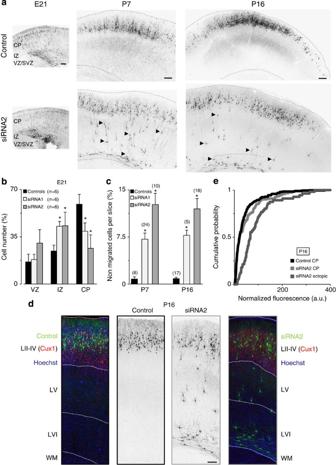Figure 2: GABAB2downregulation affects neuronal radial migrationin vivo. (a) Confocal images of tdTomato fluorescence in coronal sections of rat somatosensory cortices at different ages afterin uterotransfection (at E17) with pRNAT-U6.3 (EGFP) siRNA empty vector together with pCAG-IRES-tdTomato (Tomato, Control), or functional GABAB2-siRNA (siRNA2) together with Tomato construct (n=16–64 animals/experimental age). Arrowheads point to example neurons that did not complete radial migration. Scale bars, 200 μm. (b) Quantification of the number of neurons transfected with either siRNA vector/Tomato or control siRNAc/Tomato (controls, black) or neuron expressing either siRNA1 (light grey) or siRNA2 (dark grey), and residing at the VZ, IZ, or CP (marked by the dotted lines in a) at E21. Numbers are expressed as a percentage of the total number of fluorescent cells in the same section. Asterisks indicate statistically significant difference compared with controls (one-way ANOVA,P=0.004;post-hocHolm–Sidak method,P<0.05).n=number of rats processed (1–3 averaged slices per animal). (c) Quantification of the number of control neurons (black) or neurons expressing either siRNA1 (light grey) or siRNA2 (dark grey) that did not complete their migration at different postnatal ages. Asterisks indicate statistically significant difference compared with controls (Kruskal–Wallis one-way ANOVA,P<0.001;post-hocDunn’s method,P<0.05). Numbers in parentheses: number of rats processed (1–3 averaged slices/ per animal). (d) Confocal images of tdTomato fluorescence (green) from empty vector/Tomato- (control) or siRNA2/Tomato-transfected slices stained (at P16) for upper-layer marker Cux1 (red) and nuclear marker Hoechst (blue), showing no defects in general layering of siRNA2-transfected cortices. Dotted white lines delimitate the boundaries of the cortical layers. Scale bar, 150 μm. LII–LIV: layer II–IV; WM: white matter. (e) Cumulative distribution of the average tdTomato-fluorescence intensity at the soma in neurons transfected with control vectors (EGFP/Tomato or siRNA2/Tomato) in the CP (black and light grey, respectively) or with siRNA2/Tomato in ectopic cells (gray) was quantified as a measure of the GABAB2downregulation extent at P16. Ectopic cells exhibited higher tdTomato fluorescence intensity, consistent with severe developmental defects associated with higher levels of siRNA2 expression (Kolmogorov–Smirnov test). Figure 2b shows a quantification of the number of neurons expressing siRNA1/Tomato or siRNA2/Tomato, or either siRNA vector or siRNAc (both included in controls) residing at the VZ, IZ or CP, and normalized to the total number of transfected cells. At P7, control siRNA/Tomato cells all reached cortical layer II/III, whereas a significant percentage of the siRNA1/Tomato and siRNA2/Tomato cells were misplaced ( Fig. 2a ). Similarly, at P16 (as well as at P35) control Tomato cells were all located at cortical layer II/III, whereas a significant percentage of siRNA1/Tomato and siRNA2/Tomato cells remained in deep layers (P16: Fig. 2a P35: controls, 0.1±0.1%; siRNA2, 8.1±1.2%). Nevertheless, the general cortical layering seemed preserved, as revealed by immunostaining for the upper-layer neuron-marker Cux1 (red) and nuclear staining with Hoechst (blue, Fig. 2d ). Interestingly, we found that ectopic cells with impaired migration showed increased fluorescence-reporter expression ( Fig. 2e ), which negatively correlated with GABA B2 expression in other experiments ( Supplementary Fig. S3c ). To exclude that the defects in the radial migration may be due to a direct effect of GABA B R downregulation on radial glia fibres (radial glia is also transfected during in utero electroporation), we stained radial glia with specific marker nestin in siRNA vector/Tomato- (control) or siRNA2/Tomato-expressing animals at E21. Nestin immunostaining did not reveal any gross difference in the organization of radial glia scaffold ( Supplementary Fig. S5 ). Figure 2: GABA B2 downregulation affects neuronal radial migration in vivo . ( a ) Confocal images of tdTomato fluorescence in coronal sections of rat somatosensory cortices at different ages after in utero transfection (at E17) with pRNAT-U6.3 (EGFP) siRNA empty vector together with pCAG-IRES-tdTomato (Tomato, Control), or functional GABA B2 -siRNA (siRNA2) together with Tomato construct ( n =16–64 animals/experimental age). Arrowheads point to example neurons that did not complete radial migration. Scale bars, 200 μm. ( b ) Quantification of the number of neurons transfected with either siRNA vector/Tomato or control siRNAc/Tomato (controls, black) or neuron expressing either siRNA1 (light grey) or siRNA2 (dark grey), and residing at the VZ, IZ, or CP (marked by the dotted lines in a) at E21. Numbers are expressed as a percentage of the total number of fluorescent cells in the same section. Asterisks indicate statistically significant difference compared with controls (one-way ANOVA, P =0.004; post-hoc Holm–Sidak method, P <0.05). n =number of rats processed (1–3 averaged slices per animal). ( c ) Quantification of the number of control neurons (black) or neurons expressing either siRNA1 (light grey) or siRNA2 (dark grey) that did not complete their migration at different postnatal ages. Asterisks indicate statistically significant difference compared with controls (Kruskal–Wallis one-way ANOVA, P <0.001; post-hoc Dunn’s method, P <0.05). Numbers in parentheses: number of rats processed (1–3 averaged slices/ per animal). ( d ) Confocal images of tdTomato fluorescence (green) from empty vector/Tomato- (control) or siRNA2/Tomato-transfected slices stained (at P16) for upper-layer marker Cux1 (red) and nuclear marker Hoechst (blue), showing no defects in general layering of siRNA2-transfected cortices. Dotted white lines delimitate the boundaries of the cortical layers. Scale bar, 150 μm. LII–LIV: layer II–IV; WM: white matter. ( e ) Cumulative distribution of the average tdTomato-fluorescence intensity at the soma in neurons transfected with control vectors (EGFP/Tomato or siRNA2/Tomato) in the CP (black and light grey, respectively) or with siRNA2/Tomato in ectopic cells (gray) was quantified as a measure of the GABA B2 downregulation extent at P16. Ectopic cells exhibited higher tdTomato fluorescence intensity, consistent with severe developmental defects associated with higher levels of siRNA2 expression (Kolmogorov–Smirnov test). Full size image Thus, GABA B2 downregulation affects the radial migration of excitatory pyramidal neurons in vivo , with the strength of this effect depending on the extent of GABA B2 -protein downregulation. GABA B2 -siRNA affects axon and dendrite development in vivo Next, we investigated whether GABA B2 downregulation affected morphological maturation of siRNA2-expressing neurons. At E21, cells electroporated (at E17) with control vectors presented a different morphology depending on their location [30] . Cells residing at the SVZ, showed a characteristic stellate morphology ( Fig. 3a ) with 4–5 short processes ( Fig. 3d ). Interestingly, siRNA2/Tomato-transfected cells appeared engulfed in a net of long and thin processes ( Fig. 3b ). On the other hand, control cells at the CP presented the characteristic bipolar morphology of migrating neurons, with a leading process oriented towards the top of the cortex (the future apical dendrite), and a thin trailing process oriented towards the bottom of the cortex (the future axon; Fig. 3a ). Indeed, transition from multipolar to bipolar morphology determines the polarization of pyramidal neurons, promoting specification of one axon and multiple dendrites. Notably, siRNA2/Tomato neurons had a significantly shorter leading process than controls at the CP ( Fig. 3c ). By P16, migration of control pyramidal neurons was completed and their dendritic trees acquired complex morphology ( Fig. 3f ). However, siRNA2-transfected cells presented short and simple dendritic branching ( Fig. 3f ). Furthermore, ectopic neurons were characterized by a multipolar morphology with long and thin processes ( Fig. 3i ). 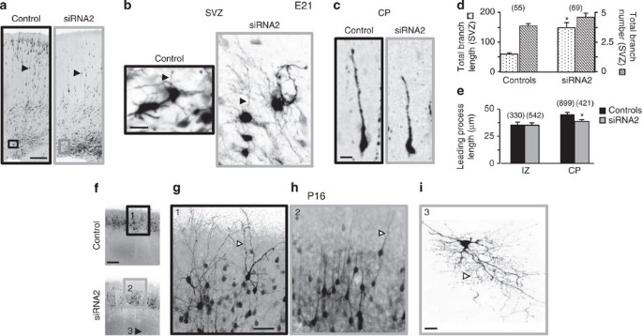Figure 3: GABAB2downregulation specifically affects axon/dendrite morphological maturation of pyramidal neuronsin vivo. (a) Confocal images of tdTomato fluorescence in coronal sections of somatosensory cortices from E21 rats transfectedin uterowith control siRNA vector/Tomato (black) or siRNA2/Tomato (grey) construct. Scale bar, 200 μm. (b) Higher magnifications of SVZ fields from boxed regions as ina. Note the abundance of long and thin processes in siRNA2-transfected cells in comparison with normal stellate morphology of SVZ control neurons (black arrowheads). Scale bar, 25 μm. (c) High-magnification images of typical bipolar migrating neurons from the CP (as indicated by arrowheads ina), showing a longer leading process in control than in GABAB2-downregulated cells. Scale bar, 10 μm. (d) Quantification of the total branch length (dots) and branch number (lines) of neurons expressing either siRNA vector/Tomato or siRNAc/Tomato (controls), or siRNA2/Tomato in the SVZ at E21. The asterisk indicates statistically significant difference compared with controls (Mann–Whitney Test,P<0.001). Numbers in parentheses: number of cells processed (control, four rats; siRNA2, six rats). (e) Quantification of the leading process length of control neurons (black), or siRNA2/Tomato (grey) at E21. The asterisk indicates statistically significant difference compared with controls (one-way ANOVA,P<0.001;post-hocHolm–Sidak method,P<0.05). Numbers in parentheses: number of cells processed (control four rats, siRNA2 six rats). (f) Confocal images of tdTomato fluorescence in coronal sections of somatosensory cortices from P16 rats transfectedin uterowith siRNA vector/Tomato (top) or siRNA2/Tomato (bottom) constructs. Scale bar, 300 μm. (g,h) Control neurons showed thick and long apical dendrites, whereas GABAB2downregulation impaired dendritic development (white arrowheads). (i) Thin and long processes (white arrowhead) were observed in ectopic cells located at deep cortical layers (as indicated by the black arrowhead inf) in siRNA2/Tomato-transfected cells. Images (g,h,i) are magnifications from square boxes inf. Scale bars: 100 μm, images 1–2; 25 μm, image 3. Figure 3: GABA B2 downregulation specifically affects axon/dendrite morphological maturation of pyramidal neurons in vivo . ( a ) Confocal images of tdTomato fluorescence in coronal sections of somatosensory cortices from E21 rats transfected in utero with control siRNA vector/Tomato (black) or siRNA2/Tomato (grey) construct. Scale bar, 200 μm. ( b ) Higher magnifications of SVZ fields from boxed regions as in a . Note the abundance of long and thin processes in siRNA2-transfected cells in comparison with normal stellate morphology of SVZ control neurons (black arrowheads). Scale bar, 25 μm. ( c ) High-magnification images of typical bipolar migrating neurons from the CP (as indicated by arrowheads in a ), showing a longer leading process in control than in GABA B2 -downregulated cells. Scale bar, 10 μm. ( d ) Quantification of the total branch length (dots) and branch number (lines) of neurons expressing either siRNA vector/Tomato or siRNAc/Tomato (controls), or siRNA2/Tomato in the SVZ at E21. The asterisk indicates statistically significant difference compared with controls (Mann–Whitney Test, P <0.001). Numbers in parentheses: number of cells processed (control, four rats; siRNA2, six rats). ( e ) Quantification of the leading process length of control neurons (black), or siRNA2/Tomato (grey) at E21. The asterisk indicates statistically significant difference compared with controls (one-way ANOVA, P <0.001; post-hoc Holm–Sidak method, P <0.05). Numbers in parentheses: number of cells processed (control four rats, siRNA2 six rats). ( f ) Confocal images of tdTomato fluorescence in coronal sections of somatosensory cortices from P16 rats transfected in utero with siRNA vector/Tomato (top) or siRNA2/Tomato (bottom) constructs. Scale bar, 300 μm. ( g , h ) Control neurons showed thick and long apical dendrites, whereas GABA B2 downregulation impaired dendritic development (white arrowheads). ( i ) Thin and long processes (white arrowhead) were observed in ectopic cells located at deep cortical layers (as indicated by the black arrowhead in f ) in siRNA2/Tomato-transfected cells. Images ( g , h , i ) are magnifications from square boxes in f . Scale bars: 100 μm, images 1–2; 25 μm, image 3. Full size image To quantify the effect of siRNA2 on dendritic trees, we performed post-hoc reconstructions of layer II/III neurons electroporated in utero with control vectors or siRNA2 and filled with biocytin through a patch clamp pipette. GABA B2 downregulation significantly reduced apical-dendrite length and branching at P16 ( Fig. 4a ). However, the biocytin-based assay did not allow analysis of axonal length because long processes were likely cut during acute-slice preparation. Therefore, for axon analyses, we used a GFP fusion protein (see Methods) that localizes at the plasma membrane (mGFP; Supplementary Fig. S2d ), which allowed visualization of neurite projections ex vivo . Thus, we coelectroporated mGFP and either siRNA vector/Tomato or siRNA2/Tomato in E17 embryos, and analysed axonal development at P16 ( Fig. 4c ). Quantification of the mGFP fluorescence intensity (normalized to the number of Tomato-positive transfected cells) at the level of dendrites ( Fig. 4c , boxed region 1) confirmed impaired dendritic development in siRNA2/Tomato animals ( Fig. 4d ). Interestingly, we found significantly higher mGFP fluorescence in layer V (axonal intra-cortical projection; Fig. 4c , boxed region 2) and white matter (WM, axonal projections to the contro-lateral cortex; Fig. 4c , boxed region 3), indicating an abnormal expansion of axonal projections in siRNA2/Tomato-transfected neurons of layer II/III ( Fig. 4d ). Similar results were obtained in animals not only at P7 (dendrites: 37±10% decrease in comparison with controls; axon layer V: 43±9% increase; axon WM: 39±11% increase; Mann–Whitney test, P <0.05), but also at P35 (dendrites: 32±8% decrease in comparison with controls; axon layer V: 49±10% increase; axon WM: 47±13% increase; Mann–Whitney test, P <0.05), indicating that the defect in morphological maturation were not due to a simple delay in developmental growth consequent to hindered migration. 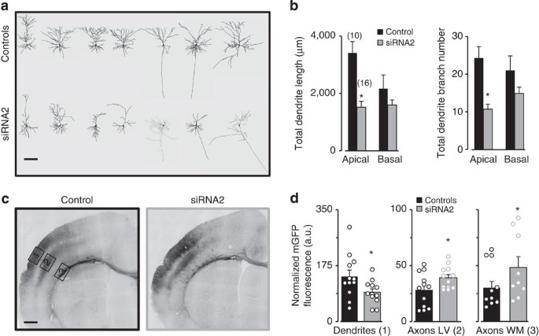Figure 4: GABAB2downregulation significantly affects axon/dendrite growth in pyramidal neuronsin vivo. (a) Neurolucida reconstruction of siRNA vector/Tomato (control) or siRNA2/Tomato pyramidal neurons filled with biocytin through a patch clamp pipette and located in layer II/III. Scale bar, 100 μm. (b) Quantification of the total dendritic length and branch number (separated for apical and basal dendrites) of all the cells reconstructed as ina. Asterisks indicate statistically significant difference compared with controls (one-way ANOVA,P<0.001;post-hocHolm–Sidak method,P<0.05). Numbers in parentheses: number of cells analysed. (c) Confocal images of the fluorescence of plasma-membrane fusion protein mGFP in coronal sections of somatosensory cortices from P16 rats transfectedin uterowith mGFP, siRNA vector and Tomato constructs (control) or mGFP, siRNA2 and Tomato constructs. mGFP allows a better visualization of dendritic trees (boxed region 1) and thin and long axonal processes with branching and projection areas in deep cortical layer V (boxed region 2) and WM (boxed region 3). Scale bar, 500 μm. (d) Quantification of total mGFP fluorescence (normalized to the number of transfected Tomato-positive cells) in fields as inc. Data points represent results from single slices (hollow circles), and the average value (±s.e.m.) is indicated by the histogram (six animals each for control and siRNA2 experiments). Data for siRNA2 were significantly different (*) from those for controls (Mann–Whitney Test,P<0.05). Figure 4: GABA B2 downregulation significantly affects axon/dendrite growth in pyramidal neurons in vivo. ( a ) Neurolucida reconstruction of siRNA vector/Tomato (control) or siRNA2/Tomato pyramidal neurons filled with biocytin through a patch clamp pipette and located in layer II/III. Scale bar, 100 μm. ( b ) Quantification of the total dendritic length and branch number (separated for apical and basal dendrites) of all the cells reconstructed as in a . Asterisks indicate statistically significant difference compared with controls (one-way ANOVA, P <0.001; post-hoc Holm–Sidak method, P <0.05). Numbers in parentheses: number of cells analysed. ( c ) Confocal images of the fluorescence of plasma-membrane fusion protein mGFP in coronal sections of somatosensory cortices from P16 rats transfected in utero with mGFP, siRNA vector and Tomato constructs (control) or mGFP, siRNA2 and Tomato constructs. mGFP allows a better visualization of dendritic trees (boxed region 1) and thin and long axonal processes with branching and projection areas in deep cortical layer V (boxed region 2) and WM (boxed region 3). Scale bar, 500 μm. ( d ) Quantification of total mGFP fluorescence (normalized to the number of transfected Tomato-positive cells) in fields as in c . Data points represent results from single slices (hollow circles), and the average value (±s.e.m.) is indicated by the histogram (six animals each for control and siRNA2 experiments). Data for siRNA2 were significantly different (*) from those for controls (Mann–Whitney Test, P <0.05). Full size image To exclude that siRNA2 transfection affected neuronal development in vivo by off-target effects, we generated a complementary DNA encoding a siRNA-resistant GABA B2 subunit (mutGABA B2 ). MutGABA B2 bore four silent mutations in the siRNA2-target sequence ( Fig. 5a ), and it was cloned into pCAG-IRES-tdTomato ( Supplementary Fig. S2g ). Co-transfection of mutGABA B2 and siRNA2 in cortical neurons in culture at days in vitro 3 (3 DIV) revealed overexpression of GABA B2 even in the presence of siRNA2 ( Fig. 5b ). In utero coelectroporation of mutGABA B2 together with siRNA2 rescued all phenotypes at P16 ( Fig. 5d–g ). Overexpression of mutGABA B2 per se did not show any effect, in agreement with previous reports indicating that fully functional GABA B Rs require coassembly of GABA B1 and GABA B2 subunits [3] . 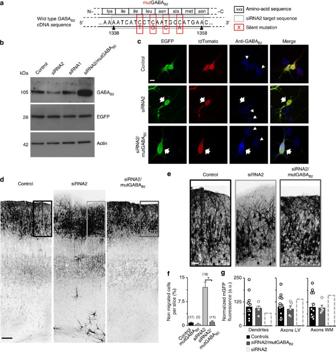Figure 5: siRNA-resistant GABAB2rescues phenotypes associated with wild-type GABAB2-subunit downregulation. (a) Cartoon exemplifying the four silent mutations (red) in the siRNA2-target sequence (grey) of the WT GABAB2cDNA (black), which confer resistance to the siRNA2 and no change in the amino-acid sequence of the resulting protein (mutGABAB2), compared with the WT. (b) Immunoblot with GABAB2subunit specific antibody on total lysate of cortical neurons (3 DIV), transfected at plating with different vectors. Note the strong expression of GABAB2subunit in cells expressing mutGABAB2, despite co-transfection with siRNA2 (seeSupplementary Fig. S10). (c) Immunostaining against GABAB2(blue) in cortical cultures (3 DIV) confirmed the strong expression of GABAB2in neurons transfected with mutGABAB2(tdTomato fluorescence), even in the presence of siRNA2 (EGFP fluorescence). Arrows point to transfected neurons; arrowheads point to endogenous GABAB2expression in non-transfected cells, for comparison. Scale bar, 25 μm. (d) Confocal images of tdTomato fluorescence in coronal sections of somatosensory cortices from P16 rats electroporatedin uteroat E17 with siRNA vector/Tomato (control), siRNA2/Tomato, and siRNA2 together with mutGABAB2-Tomato (siRNA2/mutGABAB2) constructs. Scale bar, 150 μm. (e) Higher magnifications of fields indicated ind. Scale bar, 40 μm. (f) Quantification of the number of neurons expressing either siRNA vector/Tomato or siRNAc/Tomato (controls, black), siRNA vector/mutGABAB2(light grey), siRNA2/Tomato (dark grey) or siRNA2/mutGABAB2(darkest grey) that did not complete their migration. The asterisk indicates statistically significant difference (Kruskal–Wallis one-way ANOVA,P<0.001;post-hocDunn’s method,P<0.05). Numbers in parentheses: number of rats processed (1–2 averaged slices per rat). (g) Quantification of the total mGFP fluorescence intensity (normalized to the number of transfected Tomato-positive cells and control mGFP) of dendritic branching and axonal projecting areas as inFig. 4c. The dotted rectangle represents data from siRNA-transfected cells from the experiment inFig. 4d, and reported here as a reference for the magnitude of the rescue. Figure 5: siRNA-resistant GABA B2 rescues phenotypes associated with wild-type GABA B2 -subunit downregulation. ( a ) Cartoon exemplifying the four silent mutations (red) in the siRNA2-target sequence (grey) of the WT GABA B2 cDNA (black), which confer resistance to the siRNA2 and no change in the amino-acid sequence of the resulting protein (mutGABA B2 ), compared with the WT. ( b ) Immunoblot with GABA B2 subunit specific antibody on total lysate of cortical neurons (3 DIV), transfected at plating with different vectors. Note the strong expression of GABA B2 subunit in cells expressing mutGABA B2 , despite co-transfection with siRNA2 (see Supplementary Fig. S10 ). ( c ) Immunostaining against GABA B2 (blue) in cortical cultures (3 DIV) confirmed the strong expression of GABA B2 in neurons transfected with mutGABA B2 (tdTomato fluorescence), even in the presence of siRNA2 (EGFP fluorescence). Arrows point to transfected neurons; arrowheads point to endogenous GABA B2 expression in non-transfected cells, for comparison. Scale bar, 25 μm. ( d ) Confocal images of tdTomato fluorescence in coronal sections of somatosensory cortices from P16 rats electroporated in utero at E17 with siRNA vector/Tomato (control), siRNA2/Tomato, and siRNA2 together with mutGABA B2 -Tomato (siRNA2/mutGABA B2 ) constructs. Scale bar, 150 μm. ( e ) Higher magnifications of fields indicated in d . Scale bar, 40 μm. ( f ) Quantification of the number of neurons expressing either siRNA vector/Tomato or siRNAc/Tomato (controls, black), siRNA vector/mutGABA B2 (light grey), siRNA2/Tomato (dark grey) or siRNA2/mutGABA B2 (darkest grey) that did not complete their migration. The asterisk indicates statistically significant difference (Kruskal–Wallis one-way ANOVA, P <0.001; post-hoc Dunn’s method, P <0.05). Numbers in parentheses: number of rats processed (1–2 averaged slices per rat). ( g ) Quantification of the total mGFP fluorescence intensity (normalized to the number of transfected Tomato-positive cells and control mGFP) of dendritic branching and axonal projecting areas as in Fig. 4c . The dotted rectangle represents data from siRNA-transfected cells from the experiment in Fig. 4d , and reported here as a reference for the magnitude of the rescue. Full size image Altogether, these data indicate that specific downregulation of endogenous GABA B2 in vivo leads to increased axonal growth and decreased dendritic growth. GABA B R mostly modulates cAMP signalling perinatally Next, we investigated downstream effectors of GABA B R signalling responsible for the alterations in siRNA2-transfected animals. In adult animals, GABA B Rs can decrease GABA and glutamate presynaptic release [3] . As standard in utero electroporation results in transfection of exclusively excitatory-neuron progenitors [31] , we excluded an increase in GABA release. On the other hand, we investigated whether GABA B R may modulate glutamate release perinatally (P3–7) in the somatosensory cortex of wild-type (WT) animals. We recorded glutamate-mediated spontaneous excitatory postsynaptic currents (sEPSC) before and after bath application of GABA B R antagonist CGP55845 (CGP, 2 μM, to mimic presynaptic GABA B R downregulation; Fig. 6a ). We found no difference in sEPSC frequency before and after CGP treatment ( Fig. 3b ). Conversely, CGP treatment increased sEPSC frequency at P18–19, as expected ( Fig. 6a ). 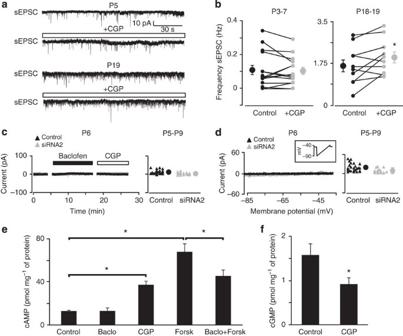Figure 6: GABABR predominantly modultes cAMP signalling during the first postnatal week. (a) Examples of glutamate-mediated sEPSC in whole-cell patch clamp recordings from neurons in layer II/III of the somatosensory cortex (recorded in bicuculline 25 μM, P5 or at −70 mV, P19) before and during bath application of GABABR antagonist CGP (2 μM). (b) Quantification of the frequencies of sEPSCs before (control) and after bath application of CGP (+CGP), recorded as ina. sEPSC frequency was increased by CGP application only at P18–19 (*, pairedt-test,P=0.04). Each symbol represents one recorded cell and the average±s.e.m. is reported on the side. Lines connect data from the same cell. (c) Examples of whole-cell patch clamp recordings showing Kir currents obtained by bath application of GABABR agonist baclofen (50 μM) and antagonist CGP (2 μM) in acute cortical slices from a WT control-(black) and a siRNA2-(grey) transfected cell at P6. The graph on the right represents the amplitude of currents measured in all recorded cells (triangles) after 10 min bath application of baclofen as in the example. The average±s.e.m. is reported on the right (circle). (d) Examples of whole-cell patch clamp recordings during a ramp test protocol (from −90 to −40 mV, 500 ms, inset) in the same set of cells as inc. The graph on the right represents the peak amplitude of baclofen-induced currents measured in all recorded cells (triangles) as in the example. The average±s.e.m. is reported on the right (circle). Peak amplitudes were calculated as inFig. 1d. (e) ELISA measurement of the cAMP level following bath application of vehicle (control), baclofen (10 μM), CGP (10 μM), forskolin (20 μM) or baclofen+forskolin to cortices acutely dissected at E17, in 5–14 independent experiments. Asterisks: statistically significant difference (One-way ANOVA,P<0.001;post-hocHolm–Sidak method,P<0.05). (f) ELISA measurement of the cGMP level following bath application of CGP (10 μM) in nine independent experiments as ine. CGP-treated cortices significantly differed (*) from controls (Mann–Whitney Test,P=0.013). Figure 6: GABA B R predominantly modultes cAMP signalling during the first postnatal week. ( a ) Examples of glutamate-mediated sEPSC in whole-cell patch clamp recordings from neurons in layer II/III of the somatosensory cortex (recorded in bicuculline 25 μM, P5 or at −70 mV, P19) before and during bath application of GABA B R antagonist CGP (2 μM). ( b ) Quantification of the frequencies of sEPSCs before (control) and after bath application of CGP (+CGP), recorded as in a . sEPSC frequency was increased by CGP application only at P18–19 (*, paired t -test, P =0.04). Each symbol represents one recorded cell and the average±s.e.m. is reported on the side. Lines connect data from the same cell. ( c ) Examples of whole-cell patch clamp recordings showing Kir currents obtained by bath application of GABA B R agonist baclofen (50 μM) and antagonist CGP (2 μM) in acute cortical slices from a WT control-(black) and a siRNA2-(grey) transfected cell at P6. The graph on the right represents the amplitude of currents measured in all recorded cells (triangles) after 10 min bath application of baclofen as in the example. The average±s.e.m. is reported on the right (circle). ( d ) Examples of whole-cell patch clamp recordings during a ramp test protocol (from −90 to −40 mV, 500 ms, inset) in the same set of cells as in c . The graph on the right represents the peak amplitude of baclofen-induced currents measured in all recorded cells (triangles) as in the example. The average±s.e.m. is reported on the right (circle). Peak amplitudes were calculated as in Fig. 1d . ( e ) ELISA measurement of the cAMP level following bath application of vehicle (control), baclofen (10 μM), CGP (10 μM), forskolin (20 μM) or baclofen+forskolin to cortices acutely dissected at E17, in 5–14 independent experiments. Asterisks: statistically significant difference (One-way ANOVA, P <0.001; post-hoc Holm–Sidak method, P <0.05). ( f ) ELISA measurement of the cGMP level following bath application of CGP (10 μM) in nine independent experiments as in e . CGP-treated cortices significantly differed (*) from controls (Mann–Whitney Test, P =0.013). Full size image In adult animals, GABA B Rs are also coupled to Kir channels. Therefore, in acute slices from animals transfected in utero , we recorded GABA B R-induced Kir currents in control WT or siRNAc-transfected cells, and siRNA2-expressing cells by bath application of GABA B R agonist baclofen (50 μM) in the presence of GABA A R (bicuculline, 2 μM), glutamate receptor (kynurenic acid, 1 mM) and voltage-gated Na + channel (tetrodotoxin (TTX), 0.1 μM) inhibitors at P5–9 ( Fig. 6c ). In control neurons, baclofen-induced K + currents were negligible in comparison with adult levels (Kruskal–Wallis one-way analysis of variance (ANOVA), Dunn’s method, P <0.05) and did not differ from currents elicited in siRNA2-transfected cells ( P <0.05; Fig. 6c ), confirming previous studies [6] . We then reasoned that cAMP may be a possible effector upon GABA B R activation at perinatal ages. Interestingly, despite large literature on GABA B R coupling to cAMP signalling in the adult neurons [3] , little evidence has been reported in young neurons [32] . To investigate this possibility in our system, we performed an ELISA immunoassay and measured cAMP levels after bath application of GABA B R agonist baclofen (10 μM, pretreatment) or antagonist CGP (10 μM) in WT rat cortices acutely dissected at E17. We used adenylyl-cyclase activator forskolin (20 μM) as positive control. We found that both CGP and forskolin treatments significantly increased cAMP levels, whereas baclofen reduced forskolin-induced cAMP increase ( Fig. 6e ). Altogether, these findings indicate that in the perinatal cortex GABA B R is negatively coupled to cAMP signalling. Thus, the defects in migration and morphological maturation of pyramidal neurons were possibly due to impairment of cAMP signalling by GABA B Rs. GABA B2 R siRNA affects in vivo neuronal development by cAMP/LKB1 cAMP is a key factor for axonal polarization and subsequent neuronal migration during perinatal development [33] , [34] , [35] , [36] . In particular, cAMP and cGMP activities transduce the action of naturally polarizing extracellular factors on axon/dendrite formation through their reciprocal regulations [35] . cAMP elevation causes cGMP decrease, promoting axon growth and specification, and suppressing dendrite formation, whereas cGMP elevation induces cAMP decrease and results in the opposite effects on axon/dendrite growth and polarization in vitro [35] . Furthermore, in vivo manipulations that increased cAMP levels, as well as manipulations that decreased cGMP levels, were all accompanied by the same phenotypes that we described above for GABA B2 -siRNA-electroporated animals [34] , [35] , [36] . Thus, we hypothesized that elevation of cAMP levels together with reduction in cGMP levels may explain developmental defects by GABA B2 downregulation. Consequently, we investigated whether cGMP level was decreased in WT rat cortices (E17) by GABA B R inhibition with CGP, due to reciprocal regulation with cAMP [35] . As expected, cAMP elevation by GABA B R inhibition was paralleled by decreased cGMP level in comparison with controls ( Fig. 6f ). Then, we assessed GABA B R involvement in cAMP/LKB1 signalling for regulation of axonal polarization in vivo . As the role of cAMP in axon initiation during neuronal polarization is regulated by phosphorylation of the downstream-kinase LKB1 at the protein kinase A (PKA)-site serine 431 (pLKB1-S431) ( [34] , [37] ), we first assessed pLKB1-S431 in E21 cortices from WT non-transfected animals. Similar to GABA B2 R expression ( Supplementary Fig. S1c ), pLKB1-S431 was highly enriched at SVZ and CP ( Fig. 7a ). Second, we investigated whether pLKB1-S431 was increased by treatment with GABA B R antagonist CGP (10 μM) in E17 WT freshly dissected cortices. We found that CGP treatment drastically increased pLKB1-S431 ( Fig. 7b ). Conversely, pretreatment with GABA B R agonist baclofen (10 μM) significantly reduced forskolin-induced increase ( Fig. 7b ). Last, we directly investigated whether siRNA2 expression in E21 neurons at the SVZ affected pLKB1-S431. We found that siRNA2 expression (green) significantly increased pLKB1-S431 immunostaining (red) in transfected neurons, in comparison with control siRNAc neurons (green) ( Fig. 7c ). 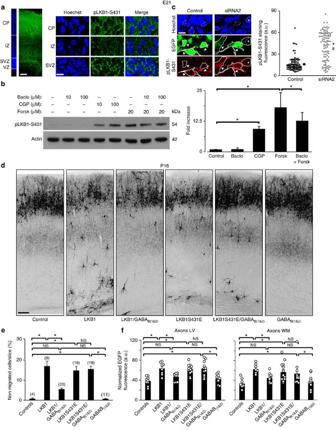Figure 7: GABABR regulates neuronal developmentin vivothrough cAMP/LKB1 signalling. (a) Left: confocal image of LKB1 phosphorylation at PKA-site serine S431 (pLKB1-S431) immunostaining (green) from a coronal section of rat somatosensory cortex at E21. Slices were counterstained with Hoechst (blue). Scale bar, 100 μm. Right: high-magnification images of SVZ, IZ and CP. Note the abundance of pLKB1-S431 in SVZ and CP. Scale bar, 10 μm. (b) Left: western blot showing pLKB1-S431, upon bath application of vehicle (control), baclofen, CGP and forskolin to cortices acutely dissected at E17 (seeSupplementary Fig. S10). Right: quantification of the fold-increase average of pLKB1-S431 compared with control, in five independent experiments as in left. GABABR inhibition by CGP (10 μM) increased pLKB1-S431, mimicking forskolin treatment (Kruskal–Wallis one-way ANOVA on ranks,P<0.001;post-hocStudent–Newman–Keuls method,P<0.05). Conversely, pretreatment with baclofen (10 μM) significantly reduced forskolin-induced pLKB1-S431 (P<0.05). (c) Confocal images of pLKB1-S431 immunostaining (red) and nucleus staining (Hoechst, blue) from a coronal SVZ section of a rat at E21 previously transfected with control siRNAc (green) or siRNA2 (green). Arrowheads point to highly transfected cells, whereas the asterisk marks a low transfected cell for comparison. Scale bar, 10 μm. Right: average cytoplasmic fluorescence measured at the cell body for all cells analysed (diamonds; three animals each per experimental case) as in the example on the left. The average±s.e.m. is reported on the right. The asterisk indicates statistically significant difference (Mann–Whitney testP<0.001). (d) Confocal images of EGFP fluorescence in coronal sections of somatosensory cortices from P16 rats transfectedin uterowith the indicated constructs. Scale bar, 150 μm. (e) Quantification of the percentage of neurons that did not complete their migration at P16 in slices from animals transfected with the indicated constructs. Asterisks indicate statistically significant difference (Kruskal–Wallis one-way ANOVA,P<0.001;post-hocDunn’s method,P<0.05). Numbers in parentheses: number of rats processed (1–2 averaged slices per animal). (f) Quantification of the average EGFP fluorescence intensity (normalized to the number of transfected Tomato-positive cells and field background) of axonal projecting areas, as inFig. 4c. NS, not significant. Figure 7: GABA B R regulates neuronal development in vivo through cAMP/LKB1 signalling. ( a ) Left: confocal image of LKB1 phosphorylation at PKA-site serine S431 (pLKB1-S431) immunostaining (green) from a coronal section of rat somatosensory cortex at E21. Slices were counterstained with Hoechst (blue). Scale bar, 100 μm. Right: high-magnification images of SVZ, IZ and CP. Note the abundance of pLKB1-S431 in SVZ and CP. Scale bar, 10 μm. ( b ) Left: western blot showing pLKB1-S431, upon bath application of vehicle (control), baclofen, CGP and forskolin to cortices acutely dissected at E17 (see Supplementary Fig. S10 ). Right: quantification of the fold-increase average of pLKB1-S431 compared with control, in five independent experiments as in left. GABA B R inhibition by CGP (10 μM) increased pLKB1-S431, mimicking forskolin treatment (Kruskal–Wallis one-way ANOVA on ranks, P <0.001; post-hoc Student–Newman–Keuls method, P <0.05). Conversely, pretreatment with baclofen (10 μM) significantly reduced forskolin-induced pLKB1-S431 ( P <0.05). ( c ) Confocal images of pLKB1-S431 immunostaining (red) and nucleus staining (Hoechst, blue) from a coronal SVZ section of a rat at E21 previously transfected with control siRNAc (green) or siRNA2 (green). Arrowheads point to highly transfected cells, whereas the asterisk marks a low transfected cell for comparison. Scale bar, 10 μm. Right: average cytoplasmic fluorescence measured at the cell body for all cells analysed (diamonds; three animals each per experimental case) as in the example on the left. The average±s.e.m. is reported on the right. The asterisk indicates statistically significant difference (Mann–Whitney test P <0.001). ( d ) Confocal images of EGFP fluorescence in coronal sections of somatosensory cortices from P16 rats transfected in utero with the indicated constructs. Scale bar, 150 μm. ( e ) Quantification of the percentage of neurons that did not complete their migration at P16 in slices from animals transfected with the indicated constructs. Asterisks indicate statistically significant difference (Kruskal–Wallis one-way ANOVA, P <0.001; post-hoc Dunn’s method, P <0.05). Numbers in parentheses: number of rats processed (1–2 averaged slices per animal). ( f ) Quantification of the average EGFP fluorescence intensity (normalized to the number of transfected Tomato-positive cells and field background) of axonal projecting areas, as in Fig. 4c . NS, not significant. Full size image If GABA B downregulation effects in vivo were the result of increased activation of cAMP/LKB1 pathway, then overexpression of GABA B R should rescue the effect of LKB1 overexpression on migration and axonal development [34] , [35] . Therefore, we performed in utero electroporation of control EGFP/Tomato, LKB1-EGFP/Tomato ( Supplementary Fig. S2e ) or LKB1-EGFP together with GABA B1 -Tomato (both isoforms B1a and B1b, Supplementary Fig. S2g ) and mutGABA B2 -Tomato (to ensure expression of a functional GABA B R), and examined the number of ectopic cells and axonal development at P16. In utero coelectroporation of two expression vectors with the same promoter resulted in coexpression of the two proteins encoded by the vectors with a tight correlation ( Supplementary Fig. S4b,d ; Pearson product moment correlation, R =0.98±0.01; n =6 animals). Overexpression of LKB1 and GABA B subunits in neurons resulted in functional proteins ( Supplementary Figs S6 and S7 ). In line with GABA B2 R downregulation, LKB1 overexpression in vivo resulted in ectopic cells and increased fluorescence in axonal-projection regions at P16 ( Fig. 7d ), as previously described [34] . Interestingly, overexpression of GABA B R (GABA B(1&2) ) together with LKB1 significantly rescued all these LKB1-induced effects. Moreover, upon expression of a constitutively active LKB1 phosphomimetic mutant at the PKA site (also affecting neuronal migration and axonal development; LKB1S431E), we found that GABA B R overexpression was not able to rescue LKB1S431E overexpression-induced defects ( Fig. 7d ). Thus, GABA B R exerted its role on LKB1 through the cAMP/PKA pathway. Conversely, GABA B(1&2) overexpression per se had no effect on migration or morphological maturation ( Fig. 7d ). That GABA B2 -siRNA affected neuronal migration and morphological maturation by LKB1 signalling was confirmed by the fact that in utero coelectroporation of LKB1-siRNA [34] and siRNA2 rescued the developmental phenotypes ( Supplementary Fig. S8 ). Altogether, these findings indicate that GABA B Rs affect migration and axonal development by modulation of cAMP/LKB1 pathway in vivo . GABA B2 R siRNA affects axon/dentrite polarization in vitro Next, we investigated whether activation of GABA B R and consequent cAMP/LKB1 signalling specifically affected axon/dendrite polarization. Unfortunately, immunostaining of abnormal processes with axon-specific markers in SVZ and ectopic multipolar siRNA2 neurons was not successful due to dense staining from non-transfected cells. Thus, we turned to cell cultures as a simplified system, as in other in vivo studies [34] , [35] , [36] , [37] , [38] . Indeed, similarly to polarization in vivo , neuronal maturation in culture undergoes polarization from a morphologically symmetric cell with multiple equivalent neurites to a polarized neuron exhibiting a single axon and multiple dendrites [30] . Therefore, we prepared primary cortical neuronal cultures and examined the effect of GABA B R modulation by treatment with GABA B R agonist baclofen (10 μM) and antagonist CGP (10 μM) 3 h after plating, or by transfection with siRNA2 at plating ( Fig. 8a ). At this stage, neurons in culture are not polarized (no axonal immunoreactivity for Smi-312, red), but exhibit multiple equivalent processes all immunopositive for GABA B2 (green, Supplementary Fig. S1e ). As positive control, we treated cultures with forskolin (20 μM). As axon/dendrite polarization is tightly linked to neurite growth [35] , we first assessed the relative length and branch numbers of axons and dendrites in treated neurons at 3 DIV, when cells have acquired a polarized morphology. Cells treated with baclofen and transfected with siRNA (EGFP) vector for visualization had longer and more branched dendrites (MAP2 staining) associated with shorter and less branched axons (Smi-312 staining; Fig. 8b ). Conversely, siRNA2 transfection or treatment with either CGP or forskolin resulted in shorter dendrites and longer axons, compared with control cells treated with vehicle (dimethylsulphoxide 0.1%) and transfected with either siRNA empty vector or siRNAc ( Fig. 8b ). 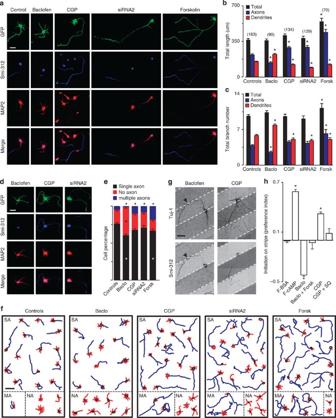Figure 8: GABAB2downregulation affects axon/dendrite growth and polarization of cortical neuronsin vitro. (a) Cultured cortical neurons (3 DIV) immunostained for axons (Smi-312, blue) and dendrites (MAP2; red). Cells were treated with vehicle (control), baclofen (10 μM), CGP (10 μM) or forskolin (20 μM) 3 h after plating, or transfected with siRNA2 at plating. All drug-treated neurons were transfected with siRNA (EGFP) vector or siRNAc for visualization. Scale bar, 50 μm. (b) Total neurite length and axonal and dendritic relative lengths of neurons as ina. Asterisks: significant difference compared with controls (one-way ANOVA,P<0.001;post-hocDunn’s method,P<0.05). (c) Total branch number and axonal and dendritic relative branch numbers of the data set inb. Asterisks: significant difference compared with controls (Kruskal–Wallis One-way ANOVA,P<0.001;post-hocDun’s method,P<0.05. (d) Neurons presenting no axon (baclofen) or multiple axons (CGP, siRNA2), following treatment as ina. Scale bar, 50 μm. (e) Percentage of neurons (four independent experiments, ~250 cells per condition) as inaandd, characterized by one single axon (black), no axon (red) and multiple axons (blue). Asterisks: significant difference compared with controls (one-way ANOVA,P<0.001;post-hocHolm–Sidak method,P<0.05). (f) Neurons reconstructed for each condition as inawith location of the cells artificially arranged for axon (blue) and dendrite (red) display. SA, single axon; MA, multiple axons; NA, no axon. Scale bar, 100 μm. (g) Neurons cultured on a substrate coated with stripes (dark grey) of baclofen (1 μM) or CGP (1 μM) and immunostained (4 DIV) for specific neuronal (Tuj-1) and axonal (Smi-312) markers. Arrowhead points to an axon turning at a baclofen stripe. Scale bar, 25 μM. (h) Preferential index (defined in the text) for axon initiation on control F-BSA (5 μg ml−1), F-cAMP (20 μM), baclofen or CGP stripes (3–4 independent experiments, ~300 cells per condition). In some experiments, forskolin (20 μM) or SQ22536 (10 μM) were bath applied to cultures. Asterisks: significant difference compared with controls (Kruskal–Wallis one-way ANOVA,P=0.016;post-hocStudent–Newman–Keuls method,P<0.05). Figure 8: GABA B2 downregulation affects axon/dendrite growth and polarization of cortical neurons in vitro . ( a ) Cultured cortical neurons (3 DIV) immunostained for axons (Smi-312, blue) and dendrites (MAP2; red). Cells were treated with vehicle (control), baclofen (10 μM), CGP (10 μM) or forskolin (20 μM) 3 h after plating, or transfected with siRNA2 at plating. All drug-treated neurons were transfected with siRNA (EGFP) vector or siRNAc for visualization. Scale bar, 50 μm. ( b ) Total neurite length and axonal and dendritic relative lengths of neurons as in a . Asterisks: significant difference compared with controls (one-way ANOVA, P <0.001; post-hoc Dunn’s method, P <0.05). ( c ) Total branch number and axonal and dendritic relative branch numbers of the data set in b . Asterisks: significant difference compared with controls (Kruskal–Wallis One-way ANOVA, P <0.001; post-hoc Dun’s method, P <0.05. ( d ) Neurons presenting no axon (baclofen) or multiple axons (CGP, siRNA2), following treatment as in a . Scale bar, 50 μm. ( e ) Percentage of neurons (four independent experiments, ~250 cells per condition) as in a and d , characterized by one single axon (black), no axon (red) and multiple axons (blue). Asterisks: significant difference compared with controls (one-way ANOVA, P <0.001; post-hoc Holm–Sidak method, P <0.05). ( f ) Neurons reconstructed for each condition as in a with location of the cells artificially arranged for axon (blue) and dendrite (red) display. SA, single axon; MA, multiple axons; NA, no axon. Scale bar, 100 μm. ( g ) Neurons cultured on a substrate coated with stripes (dark grey) of baclofen (1 μM) or CGP (1 μM) and immunostained (4 DIV) for specific neuronal (Tuj-1) and axonal (Smi-312) markers. Arrowhead points to an axon turning at a baclofen stripe. Scale bar, 25 μM. ( h ) Preferential index (defined in the text) for axon initiation on control F-BSA (5 μg ml −1 ), F-cAMP (20 μM), baclofen or CGP stripes (3–4 independent experiments, ~300 cells per condition). In some experiments, forskolin (20 μM) or SQ22536 (10 μM) were bath applied to cultures. Asterisks: significant difference compared with controls (Kruskal–Wallis one-way ANOVA, P =0.016; post-hoc Student–Newman–Keuls method, P <0.05). Full size image Furthermore, to address whether GABA B R signalling modulates axonal specification, we quantified the number of cells with one axon (SA), no axon (NA) or multiple axons (MAs) in cortical cultures ( Fig. 8d ). The percentages of SA, NA and MA cells in control conditions were 76.2±1.4%, 18.6±1.3%, 5.1±0.2%, respectively ( Fig. 8e ). Interestingly, bath application of baclofen strongly increased the percentage of NA cells and decreased the percentage of MA cells ( Fig. 8e ). Conversely, bath application of either CGP or forskolin, or siRNA2 transfection, increased the percentage of MA cells ( Fig. 8e ). Figure 8f represents samples of reconstructed neurons from drug-treated cultures. To address whether GABA B R signalling specifically affected axonal initiation, we prepared cortical cultures plated on stripe substrates of a membrane-permeable fluorescent analogue of cAMP (F-cAMP, 20 μM), GABA B R agonist baclofen (1 μM, together with fluorescent bovine serum albumin (F-BSA; 5 μM) antagonist CGP (1 μM, with F-BSA) or control GABA B R F-BSA, which is a well-established method for studying axonal specification [34] , [35] , [36] , [38] . Immunostaining of neurons at 4 DIV with axon-marker Smi-312 and neuronal marker Tuj-1 ( Fig. 8g ), revealed that for all polarized neurons with the cell body located at a stripe boundary, the presence of GABA B R agonist baclofen resulted in a large increase of axon initiation off the baclofen stripe, as exemplified by the high preference index (PI, defined as ((% on stripe)—(% off stripe))/100; Fig. 8h ). Notably, some axons revealed growth repulsion from baclofen stripes, as previously reported for cGMP stripes [34] , [35] ( Fig. 8g ). Conversely, polarized neurons with the cell body located at the boundary of either CGP or F-cAMP stripes exhibited large axon initiation on the stripes. Interestingly, a causal link between GABA B R and cAMP decrease was demonstrated by the fact that the PI returned to control levels when cell cultures on baclofen stripes were treated with forskolin (20 μM; Baclo+Forsk) or when cell cultures on CGP stripes were treated with adenylyl-cyclase inhibitor SQ22536 (10 μM; CGP+SQ; Fig. 8h ). Altogether, these data are in agreement with the in vivo experiments and identify GABA B R as a modulator of axon/dendrite growth and polarization by inhibition of cAMP signalling. Here, we coupled siRNA to in utero electroporation to downregulate endogenous GABA B2 in a subpopulation of newly born cortical neurons and determine in vivo function of this receptor for neurons in their native environment. We found that GABA B2 downregulation in vivo impaired radial migration and morphological maturation of cortical neurons by modulation of cAMP/LKB1 pathway. Our in vitro studies demonstrated that the specific morphological effects on axon and dendrites derived from a defect in neuronal polarization. Developing neural tissues are enriched in GABA [1] , [2] . In particular, as interneurons migrate tangentially in cortical IZ, GABA-positive cells increase in number and establish gradients of secreted GABA that migrating excitatory neurons sense through GABA A ( [6] ), but possibly also GABA B receptors ( Supplementary Fig. S9 ). GABA concentration in the developing brain remains even higher due to immature blood–brain barrier [39] and re-uptake system [40] , leading to tonic activation of GABA A Rs [29] . Interestingly, tonic GABA A ergic signalling is not hyperpolarizing but depolarizing and mostly excitatory during development [1] , [2] , [4] , and glutamatergic-system development lags behind. This allows to excite developing neurons for maturation, while avoiding the toxic effects of a mismatch between GABAergic inhibition and glutamatergic excitation [7] . Here, we showed that also GABA B R signalling is not hyperpolarizing in early development, in keeping with above. Moreover, we indirectly provided evidence that also GABA B Rs are under tonic activation by endogenous GABA at this age. Indeed, despite the abundance of GABA B R that we and others found in the cortex [8] , [32] , application of GABA B R agonist baclofen to embryonic cortices did not decrease basal level of cAMP and pLKB1-S431. Conversely, blockade of endogenous GABA B R by antagonist CGP revealed a significant effect. We hypothesize that the lack of baclofen effect on basal cAMP and pLKB1-S431 was due to high concentration of endogenous GABA in the developing tissue that may tonically saturate GABA B R responses, conversely, unmasked by CGP application. Accordingly, in cell cultures (10% of GABAergic interneurons; Supplementary Fig. S1d ) where endogenous GABA concentration is likely diluted by the cell medium, baclofen generated larger effects than CGP treatment or siRNA2 transfection. This is demonstrated by the fact that: (1) baclofen treatment affected both axonal length and branch number, whereas CGP treatment or siRNA2 transfection affected axonal length only. (2) Baclofen treatment affected MA and NA cell populations, whereas CGP treatment or siRNA2 transfection affected MA population only. (3) Baclofen stripes occasionally induced a repulsion effect for axonal growth, whereas the predicted attraction effect was never found for CGP stripes. (4) PI of axon initiation for repulsive baclofen stripes was ~1.5 fold larger than that for attractive CGP stripes. Despite some contrasting results by few previous studies, there is general agreement that GABA B R signalling affects axonal growth and modulates neuronal migration in vitro [9] , [10] . In particular, in line with our data, GABA B R antagonist delayed migration of excitatory neurons from the IZ to the CP [17] , and produced accumulation of tangentially migrating interneurons (associated with a shorter leading neuronal process) in the VZ/SVZ of organotypic cortical slices independently of Kir channels [15] . Conversely, in vivo studies in a number of genetically modified mice with targeted deletion or upregulation of GABA B1 or GABA B2 indicated no gross brain-morphology abnormalities [6] . The defects in GABA B R-downregulated neurons seen here and in the in vitro literature may depend on the different experimental manipulations and knockdown timing. Indeed, delivery of siRNA in utero at E17 or in cell cultures at 0 DIV versus life-long deletion or long-term overexpression of GABA B Rs in genetically modified mice may favour compensatory mechanisms in the latter case. Additionally, one must distinguish between manipulations of the global network (GABAergic system included) in genetically modified mice, versus manipulations in individual excitatory neurons within a normally developing network, as in our study. Finally, developmental defects in GABA B R genetically modified mice may have been simply overlooked due to in vivo system complexity. Indeed, the epileptic phenotype observed in adult mice knockout for the GABA B1 subunit (lacking the inhibitory hyperpolarization by GABA B activation of Kir3.2) is more severe than that observed in the weaver mouse (mutated Kir3.2 channels) or in the Kir3.2 knockouts [19] , [41] , [42] , [43] . This suggested that GABA B R modulation of downstream effectors other than Kir3.2 channels may provide a critical component of GABA B R signalling during development [20] , [41] , [44] , as confirmed here for cAMP/LKB1 pathway. We found that GABA B R mainly regulates cAMP levels during early development. We concluded that GABA B R is a modulator of neuronal polarization in vivo through cAMP/LKB1 pathway based on the following evidence: (1) in vitro GABA B2 downregulation affected axon/dendrite growth and polarization by cAMP pathway; (2) in vivo defects due to GABA B2 -siRNA phenocopied the effects upon increase of cAMP/LKB1 signalling in vivo [34] , [35] , [36] , (3) in vivo GABA B R overexpression significantly rescued LKB1- (but not phosphomimetic LKB1-S431E) overexpression effects. Accordingly, GABA (through GABA B R signalling) shares similarities with polarization molecules. First, GABA B R is abundantly expressed at the level of the VZ/SVZ, where neuronal polarization takes place. Second, like other polarizing molecules (for example, TGFβ) [38] , GABA is possibly expressed in a steep gradient (above the SVZ) by GABAergic cells tangentially migrating in the cortex ( Supplementary Fig. S9 ). However, in strong contrast with active determinants [33] of neuronal polarization (for example, LKB1), which in vitro show axonal-fate predictive-accumulation in one single process at a time when neurons are yet not polarized [34] , GABA B R showed similar expression in all non-polarized neurites in cultured neurons. We hypothesize that at SVZ, in unpolarized neurons expressing GABA B R equally in all neurites, the process facing the CP (future dendrite) be more likely to sense higher concentration of GABA translated in low cAMP level by GABA B Rs. Thereby, GABA B R would inhibit axonal formation by low cAMP, while favoring dendrite formation by high cGMP level ( Supplementary Fig. S9 , inset) [35] . Thus, beside determinants of neuronal polarization (for example, LKB1) and natural polarizing factors [33] (for example, neurotrophins, semaphorins), we postulate in vivo the existence of molecules such as GABA that simply modulate [33] the polarization process due to specific temporal (for example, GABA released from migrating interneurons at E18) and spatial (migrating interneurons located above polarizing excitatory cells) cues ( Supplementary Fig. S9 ). The hypothesis that GABA B R signalling may act as a modulator [33] , rather than a determinant of neuronal polarization in vivo is further strengthened by the fact that, while overexpression of LKB1 lead to defective polarization in vivo , overexpression of GABA B subunits did not. This indicates that the gradient generated by the migrating interneurons may possibly be the ultimate responsible for the polarization effect in GABA B2 -siRNA animals. Thus, proper development of neural network in vivo may indeed require accumulation of active determinants of neuronal polarization [33] (for example, LKB1) at the bipolar stage, but with respect to coordinates by external cues in the surrounding tissue (for example, GABA from migrating interneurons) modulating final polarization commitment [45] . Therefore, we cannot exclude that at other stages or in other brain regions characterized by different cellular environments GABA B R activation may be functional to different developmental processes. Is the defect in neuronal polarization also important for migration of newborn neurons? As neuronal polarization in vivo occurs before radial migration, migration defects may be attributed in part to the axonal polarization defect in GABA B -siRNA cells, as already hypothesized in other studies [34] , [35] , [36] , [46] . In support of this idea, we note that only cells displaying bipolar morphology were located at the CP for GABA B2 -siRNA neurons, and that these cells also expressed lower levels of GABA B2 -siRNA. Moreover, ectopic neurons were the most morphologically affected. However, we cannot exclude that failure in radial migration may be due to the reduced length in apical dendrites. Finally, we indicate cAMP/LKB1 signalling as responsible for the described effects on newborn cortical neurons. However, we cannot exclude the participation of some of the other signalling pathways downstream of GABA B R [34] , [47] , [48] , [49] , [50] , [51] . In conclusion, our study revealed an unknown function for GABA B R through cAMP/LKB1 pathway during early cortical development. This drives attention on possible side effects of the clinical use of centrally acting drugs such GABA B R agonist baclofen (a myorelaxant and painkiller) or substances that increase extracellular levels of GABA (many antiepileptics) in pregnant women and children. Generation of siRNAs and plasmid constructs We generated two 21-oligonucleotide siRNA duplexes targeting rat GABA B2 subunit (starting position: 1,338, seq no. 1; 975, seq no. 2). For mutGABA B2 vector, we created a siRNA-resistant GABA B2 cDNA by introducing four silent mutations in the siRNA2-target sequence of rat GABA B2 cDNA (gift of Dr Kaupmann, Novartis Pharma AG, Basel; NM_031802) with the QuickChange lightning mutagenesis kit (Stratagene, La Jolla, CA). PCR-based strategies were used to generate the serine-to-glutamic acid point mutation of LKB1 at the PKA-site Ser431 (LKB1S431E). Lymphocyte-specific-kinase membrane-anchor domain (aLCK)-GFP vector (gift of Dr Canossa), allowed expression of aLCK-GFP fusion protein that localizes at the plasma membrane (mGFP), and was used for better visualization of thin neuronal processes in vivo . In utero electroporation Timed-pregnant Sprague Dawley rats (Harlan Italy SRL, Correzzana, Italy) were anaesthetized at E17 with isoflurane (induction, 3.5%; surgery, 2.5%), and uterine horns were exposed by laparotomy. Expression vectors (1–2 μg μl −1 /Vector in water) and dye Fast Green (0.3 mg ml −1 ; Sigma, St. Louis, MO) were injected (5–6 μl) through the uterine wall into one of the embryos’ lateral ventricles by a 30-G needle (Pic indolor, Grandate, Italy). Each embryo’s head was held between tweezer-type electrodes (10 mM diameter; Nepa Gene, Chiba, Japan) across the uterus and five electrical pulses (amplitude, 50 V; duration, 50 ms; intervals, 100 ms) were delivered with a square-wave electroporation generator (CUY21EDIT; Nepa Gene). Uterine horns were returned into the abdominal cavity, and embryos continued their normal development. For later identification, control embryos were injected in the left ventricle, whereas experimental embryos in the right ventricle. Experiments were approved by IIT licensing and Italian Ministry of Health. Slice histology E18–P1 brains were directly fixed in 4% paraformaldehyde (PFA in PBS). P2–P16 brains were fixed by transcardial perfusion of 4% PFA. Brains were sectioned coronally 80-μm thick with a vibratome (Leica VT1000S). Free-floating slices were permeabilized and blocked with PBS containing 0.3% Triton X-100, 10% NGS and 0.2% BSA. Primary antibodies were incubated in PBS containing 5% NGS and 0.1% BSA (guinea pig anti-GABA B2 1:1,500 (Millipore, Billerica, MA); rabbit anti-GABA 1:1,000 (Sigma); rabbit anti-pLKB1-S431 1:100 (Santa Cruz) with peptide-LKB1 preincubation (1:50, 30 min)). Immunostaining was detected using Alexa fluorescent secondary antibody 1:600 (Invitrogen) in PBS containing 5% NGS. Slices were counterstained with Neurotrace Nissl 640/660 (1:100; Invitrogen Corporation, Carlsbad, CA) or Hoechst (2.5 μg μl −1 ; Sigma). Samples were mounted in Vectashield (Vector Laboratories, Inc., Burlingame, CA) and examined with confocal microscopy. For biocytin experiments, we used 400-μm-thick acute slices from patch clamp recordings where biocytin (3–4 mg ml −1 , Sigma) was added in the pipette solution. Slices were fixed in 4% PFA. Revelation of biocytin-injected neurons was obtained with Vectastain ABC Elite kit (Vector Laboratories), and slices were mounted in Mowiol (Calbiochem, La Jolla, CA). Biocytin-filled neurons were drawn by using a camera lucida (Olympus, Düsseldorf, Germany) and were computer reconstructed and analysed using Neurolucida and Neurolucida explorer (MicroBrightField, Colchester, VT). Confocal and Neurolucida image acquisition and analysis For analysis of migration at E21–P16, images from sections counterstained with Neurotrace Nissl 640/660 or Hoechst staining were acquired on a confocal laser-scanning microscope (TCS SP5; Leica Microsystems, Milan, Italy) equipped with a × 10 immersion objective (numerical aperture (NA) 0.3). Confocal images (15-μm-thick z -stacks) were acquired, and Z -series were projected to two-dimensional representations. The contrast of the images was adjusted to enhance the fluorescence of cell bodies, while attenuating the signal from neuronal processes to facilitate cell counting. For quantification of non-migrating cells, all cells in the VZ/SVZ, IZ or CP were counted and normalized to the total number of cells in the slice. Two-three slices were acquired for each animal and averaged together. For high-magnification images of cell morphology, 80-μm-thick z -stacks were acquired with a × 63 immersion objective (NA 1.4), and Z -series were projected to two-dimensional representations. In some experiments, we took advantage of mGFP fusion protein (for quantification of neurite processes) and transfected it together with Tomato (for counting of the number of transfected cells). For mGFP ( Figs 4 and 5 , Supplementary Fig. S8 ) or EGFP ( Fig. 7 ) quantification of axons and dendrites, six confocal images/slice (one single focal plane for both mGFP and tdTomato fluorescence at the level of brightest tdTomato fluorescence) were acquired (× 10 objective, NA 0.4, or × 20 objective, NA 0.5) for fields at the layer II/III, layer V and white matter (as indicated in Fig. 4 ) of transfected animals. Total mGFP or average EGFP fluorescence was calculated for each field with the Leica LAS AF Lite software (Leica Microsystems for fluorescence), and normalized to the total number of transfected (tdTomato) positive (mGFP, EGFP) cells and to slice background (EGFP). For cell-culture experiments, confocal images (one single focal plane at level of the brightest EGFP fluorescence) were acquired with a × 40 immersion objective (NA 1.25). For each litter of animals or cell-culture experiment, all slides were acquired in a random order and in a single session to minimize errors caused by fluctuation in laser output and degradation of fluorescence. For correlation analysis of different fluorescence level in slices ( Fig.2 ; Supplementary Fig. S4 ), cells were acquired with a × 40 immersion objective (one single focal plan at the level of brightest tdTomato fluorescence, for cells at CP and ectopic neurons). All experiments were acquired and analysed in a blind manner. Electrophysiology Coronal somatosensory cortical slices were acutely isolated from rats (400 μm thick) in ice-cooled cutting solution with the following composition (in mM): 0.1 MgCl 2 ; 2.5 KCl; 1.25 NaH 2 PO 4 ; 2 MgSO 4 ; 0.1 CaCl 2 ; 26 NaHCO 3 ; 206 sucrose and 12 D -glucose (~300 mOsm, pH 7.4), oxygenated with 95% O 2 and 5% CO 2 . Slices were incubated in artificial cerebrospinal fluid (ACSF) with the following composition (in mM): 124 NaCl; 2.5 KCl; 1.25 NaH 2 PO 4 ; 2 MgSO 4 ; 2 CaCl 2 ; 26 NaHCO 3 and 12 D -Glucose (~310 mOsm, pH 7.4), oxygenated with 95% O 2 and 5% CO 2. After 1-h recovery, slices were used under continuous perfusion of ACSF at room temperature. Whole-cell patch clamp recordings were made with a Multiclamp 700B amplifier (Molecular Devices). Data were sampled at 20 KHz, filtered at 5 KHz, and analysed off-line with Clampfit software (Molecular Devices). Cell culture and transfection In neuronal cell-culture experiments, cell density was 25,000 cells per cm 2 for immunostaining experiments, and 7,500 cells cm −2 for stripe experiments ( Supplementary Information ). Primary cultures of dissociated cortical neurons were prepared from E18 rat embryos and maintained in Neurobasal medium supplemented with: 2% B-27 supplement, 0.5 mM glutamine, 50 μg ml −1 of penicillin and 50 μg ml −1 of streptomycin (Invitrogen). For measurements of neurite or axon/dendrite lengths, and SA MA and NA classification, cells were treated with forskolin (20 μM), baclofen (10 μM), CGP55845 (10 μM), SQ22536 (10 μM) starting 3 h after plating, and drugs were present throughout the duration of the experiment. Cells (4 × 10 6 ) were transfected before plating by electroporation with Amaxa basal nucleofector kit for primary neurons (Lonza; transfection efficiency=80–90% of total neurons) by 3–4 μg of plasmid DNA in the Amaxa nucleofector device (program 003) according to the manufacturer’s protocol. Immunostaining For immunostaining, neurons were fixed with 4% PFA in PBS for 15 min, followed by 15-min treatment with 0.1% Triton X-100, and 2 h blocking with 10% NGS. Primary antibodies (guinea pig anti-GABA B2 1:1,500 (Millipore); rabbit anti-GABA 1:1,000 (Sigma); rabbit anti-MAP2 1:3,000 (Covance, Research Products, Inc., Berkeley, CA); mouse anti-Smi-312 1:800 (Covance); chicken anti-βIII tubulin 1:1,000 (Millipore)); rabbit anti-pLKB1-S431 1:100 (Santa Cruz) with preincubation of LKB1 peptide (1:50, 30 min); mouse anti-Nestin 1:100 (Abcam); rabbit anti-CDP (Cux1) 1:100 (Santa Cruz) were incubated in PBS containing 5% NGS. Fluorescently conjugated secondary antibodies (Alexa 488, Alexa 568 and Alexa 647 at 1:1,000, or CY5 at 1:100 (Jackson ImmunoResearch Laboratories, West Grove, PA, USA)) were incubated in PBS containing 5% NGS. Samples were counterstained with Hoechst (2.5 μg μl −1 ), mounted in Vectashield (Vector Laboratories, Inc., Burlingame, CA), and examined with confocal microscopy (see above), followed by neurite tracing and quantification with the NeuronJ plugin of ImageJ software (NIH, http://rsb.info.nih.gov/ij/ ) [52] . cAMP and cGMP measurements Levels of cAMP and cGMP in rat freshly dissected cortices (E17) were measured with cAMP and cGMP EIA kits (Cayman Chemical). After 2 h recovery in ACSF oxygenated with 95% O 2 and 5% CO 2 , baclofen and CGP were preincubated (15 min, room temperature) before bath application of forskolin (15 min). Statistical analysis Statistical analysis was performed with Student’s t- test or one-way ANOVA and post-hoc comparison. For datasets of non-normal distribution, Mann–Whitney rank sum test or Kruskal–Wallis one-way ANOVA on ranks test was used. All average data were presented as mean±s.e.m. The label ‘Control’ was used when a single example was reported in the figure, whereas ‘Controls’ was reported in summary graphs with averages. ‘Controls’ indicated that diverse types of controls were averaged (that is, cell transfected with empty vector, cells transfected with scramble siRNA, WT cells) after an appropriate statistical test established no differences among them. How to cite this article: Bony, G. et al . Non-hyperpolarizing GABA B receptor activation regulates neuronal migration and neurite growth and specification by cAMP/LKB1. Nat. Commun. 4:1800 doi: 10.1038/ncomms2820 (2013).